A far-off-resonance optical trap for a Ba+ion Optical trapping and ions combine unique advantages of independently striving fields of research. Light fields can form versatile potential landscapes, such as optical lattices, for neutral and charged atoms, while avoiding detrimental implications of established radiofrequency traps. Ions interact via long-range Coulomb forces and permit control and detection of their motional and electronic states on the quantum level. Here we show optical trapping of 138 Ba + ions in the absence of radio-frequency fields via a far-detuned dipole trap, suppressing photon scattering by three orders of magnitude and the related recoil heating by four orders of magnitude. To enhance the prospects for optical as well as hybrid traps, we demonstrate a method for stray electric field compensation to a level below 9 mV m −1 . Our results will be relevant, for example, for ion–atom ensembles, to enable 4–5 orders of magnitude lower common temperatures, accessing the regime of ultracold interaction and chemistry, where quantum effects are predicted to dominate. Trapping of ions was demonstrated decades earlier than trapping of neutral atoms, although the concepts are closely related [1] , [2] . A prominent reason is the much higher well depth provided by radio-frequency (rf) traps, on the order of 10 4 K, compared with traps for neutral particles. Optical dipole traps, for example, typically provide depths in the 10 −3 K range. The discrepancy is mainly due to the comparatively large Coulomb forces that can be exerted on charged particles. Over many years, independent research on trapped ions and atoms has seen a remarkable growth of knowledge [3] , [4] advancing various topics, for example, quantum information [5] , [6] and quantum metrology [7] , [8] , [9] , [10] , [11] , or cold collisions [12] , related to chemistry and astrophysics. The advantages related to the charge of the ions, such as the unique controllability of electronic and motional degrees of freedom on the quantum level and their characteristics to mediate long-range interactions, come at the price of their high sensitivity to stray electric fields. In rf traps, these fields displace the ion from the node of the rf potential and result in an rf-driven oscillation, the so-called micromotion [1] . Several techniques have been developed to compensate stray electric fields [13] , [14] , [15] , [16] , [17] , [18] , [19] . Nevertheless, residual rf micromotion still limits the progress in several fields of research. For example, in metrology the related second-order Doppler shift contributes significantly to the inaccuracy of atomic clocks [7] , [9] . Further improving the compensation is crucial. However, a fundamental impact of the rf field, even in the absence of any stray electric field, has been revealed recently [20] for the intriguing experiments carried out in hybrid traps [21] , [22] , [23] , [24] , [25] , [26] . In this approach, trapped neutral atoms or molecules are spatially overlapped with an ion or ions confined in an rf trap. Even if the ion is additionally considered as a classical point-like particle at zero temperature at the minimum of the rf potential, the polarization induced in an approaching atom in turn leads again to a displacement of the ion. This results in the rf field acting as a driving perturbation in the ion–atom ensemble, effectively pumping energy into the system. It has been shown that the common equilibrium temperature is not determined by the cold atomic bath (for Rb ~100 nK), but limited by the rf drive to the millikelvin regime [20] . Replacing rf fields and confining ions optically is predicted to be advantageous in several applications: to open up novel prospects in extended potential landscapes, such as optical lattices, for arrays of ions [27] or for exploiting the advantages of trapping atoms and ions simultaneously [28] , [29] , [30] , [31] and to circumvent rf micromotion by omitting any rf fields [20] . We will emphasize the latter as one showcase and consider its potential impact on the field of ultracold chemistry. Here, embedding ions optically in quantum degenerate gases is predicted to allow reaching temperatures 4–5 orders of magnitude below the current state-of-the-art [20] . In this temperature regime quantum effects are expected to dominate, in many-body physics, including the potential formation and dynamics of mesoscopic clusters of atoms of a Bose–Einstein condensate (BEC), binding to the ‘impurity ion’ [32] . At the same time, quantum effects should also dominate in two-particle s-wave collisions, the ultimate limit in ultracold chemistry [12] , [20] , [33] . Recently, optical trapping of a single ion has been demonstrated, first in a single-beam dipole trap, superimposed by a static electric potential [34] , [35] . Subsequently, all-optical trapping of an ion in an optical lattice (one-dimensional standing wave) has been achieved [36] . In these proof-of-principle experiments, the frequency of the dipole laser has been tuned close to the relevant transition, severely compromising the performance of the trap by the off-resonant scattering of photons. In addition, optical confinement in one dimension has been reported, pinning an ion or suppressing ion transport in a hybrid trap. Radially, the ion(s) remain confined along two axes by an active linear rf trap, while the third is overlapped with a far off-resonant [37] and near-resonant, blue detuned [38] , standing wave of an optical cavity, respectively. In this work, we show optical trapping of a 138 Ba + ion in the absence of rf fields in a far-off-resonance optical trap, suppressing photon scattering by three orders of magnitude and the related recoil heating by four orders of magnitude. To enable the prospects of experiments in optical as well as in hybrid traps, we propose and implement a generic method for sensing and compensating stray electric fields, currently to a level below 9 mV m −1 . Optical trapping of Ba + in a far-off-resonance dipole trap The protocol for optical trapping is illustrated in Fig. 1 . We still exploit an rf trap [39] , [40] (depicted in Fig. 1a ) to load [41] , cool and finally detect the ion. In addition, we use the rf field to trap an ion for sensing and compensating stray electric fields and to optimize the spatial overlap of the rf and the optical trap. The latter is essential for an efficient transfer. We start the optical ion-trapping sequence by switching off the cooling beam (transition between the electronic states | S 1/2 ›←| P 1/2 › at 493 nm) and subsequently the repumping beam (| D 3/2 ›←| P 1/2 › at 650 nm) to prepare the ion in the electronic ground state | S 1/2 ›. We increase the power of the dipole trapping beam (at 532 nm) linearly to its level P . After turning off the voltage supply of the rf trap, we electronically disconnect it. In the subsequent time span Δ t the ion is trapped by optical means assisted by carefully chosen and oriented d.c. fields. After turning on the rf trap and turning off the dipole trap, we employ resonant fluorescence detection to reveal if the optical trapping attempt has been successful. 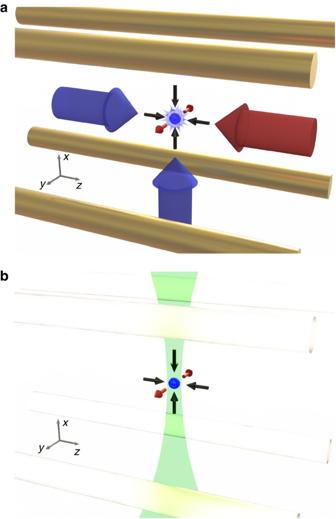Figure 1: Schematic of the setup and the optical ion-trapping sequence. (a) We start by Doppler cooling the ion from two directions (blue arrows, from left and bottom) and repumping (red arrow, from right) from one direction in a linear rf trap (depicted as four quadrupole electrodes; not to scale). After carrying out a coarse compensation of stray electric fields (see Methods), we turn off the cooling lasers followed by the repumping laser to assure pumping into the electronic ground state |S1/2›. The d.c. potential is chosen to be defocusing along theyaxis, but focusing along thez- andx-axes, symbolized by the outwards (red) and inwards (black) pointing arrows, respectively. The distorted shape surrounding the ion symbolizes its driven rf micromotion, superimposed on the harmonic motion within the time-averaged trapping potential. (b) We turn on the dipole trapping laser (green) and switch off the rf trap (the deactivated rf drive is indicated by the translucent electrodes). That is, we provide confinement by optical dipole and d.c. potentials only. After a duration Δt, we turn on the rf trap, the cooling and the repumping laser again while we turn off the dipole trapping laser. In the case of successful optical trapping, we finally detect the ion with a CCD camera via resonant fluorescence in the rf trap (seea). Figure 1: Schematic of the setup and the optical ion-trapping sequence. ( a ) We start by Doppler cooling the ion from two directions (blue arrows, from left and bottom) and repumping (red arrow, from right) from one direction in a linear rf trap (depicted as four quadrupole electrodes; not to scale). After carrying out a coarse compensation of stray electric fields (see Methods), we turn off the cooling lasers followed by the repumping laser to assure pumping into the electronic ground state | S 1/2 ›. The d.c. potential is chosen to be defocusing along the y axis, but focusing along the z - and x -axes, symbolized by the outwards (red) and inwards (black) pointing arrows, respectively. The distorted shape surrounding the ion symbolizes its driven rf micromotion, superimposed on the harmonic motion within the time-averaged trapping potential. ( b ) We turn on the dipole trapping laser (green) and switch off the rf trap (the deactivated rf drive is indicated by the translucent electrodes). That is, we provide confinement by optical dipole and d.c. potentials only. After a duration Δ t , we turn on the rf trap, the cooling and the repumping laser again while we turn off the dipole trapping laser. In the case of successful optical trapping, we finally detect the ion with a CCD camera via resonant fluorescence in the rf trap (see a ). Full size image To derive the dependency of the optical trapping probability on the depth of the total potential U tot (optical and d.c. confinement), we first confirm that the cooling, repumping, stray field compensation and beam alignment are set appropriately. For this purpose, we perform one test at the maximum trap depth U max ≈ k B × 62 mK, k B denoting the Boltzmann constant, achieved with a trapping laser power of P max ≈13.1 W at a beam waist W =3.9 μm (1/ e 2 of the intensity I ). The average of all performance tests amounts to (89±4) % and is depicted in Fig. 2 . Subsequently, we decrease the power of the dipole laser to P , corresponding to one specific trap depth U tot , and repeat the trapping sequence to determine the optical trapping probability P trap with a statistical uncertainty of <10% (1 σ ). The results for one specific set of parameters are shown in Fig. 2 (blue filled circles). For P =0 W ( U tot = k B × 0 K), P trap is zero, demonstrating that residual trapping fields remain negligible and confinement in three dimensions for P >0 W is achieved by means of optical dipole forces. We fit the measured data with a model function and derive an initial ion temperature T init =(8.5±0.7) mK (see Methods). 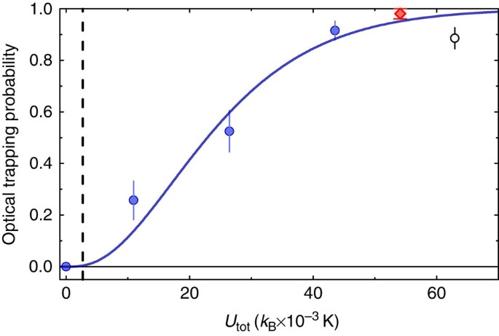Figure 2: Optical trapping probability in dependence on the total trap depthUtot. For eachUtot, controlled by the power of the dipole laser beam, we prepare the ions in the rf trap (seeFig. 1a), compensate stray electric fields and run a performance test at maximal optical trap depth,Umax≈kB× 62 mK (black open circle). Subsequently, we reduceUtotto one of four values (blue filled circles). Under optimized conditions (see text), we observe improved probabilities for optical trapping (red diamond). We choose a trapping duration sufficiently short (Δt=100 μs) to avoid shelving into the |D› manifolds currently limiting the lifetime atUmaxto milliseconds. To demonstrate optical trapping, we compensate the stray electric field to a level of ~80 mV m−1only. The corresponding electric force results in a threshold for the critical optical potentialUcritdepicted as the vertical dashed line. Applying our novel compensation method to its current limitation of 8.7 mV m−1(see text) will allow us to further reduce the laser power of the dipole beam and to increase the lifetime of the ion substantially. The vertical error bars denote the statistical error (1σ) of the respective measurement. Figure 2: Optical trapping probability in dependence on the total trap depth U tot . For each U tot , controlled by the power of the dipole laser beam, we prepare the ions in the rf trap (see Fig. 1a ), compensate stray electric fields and run a performance test at maximal optical trap depth, U max ≈ k B × 62 mK (black open circle). Subsequently, we reduce U tot to one of four values (blue filled circles). Under optimized conditions (see text), we observe improved probabilities for optical trapping (red diamond). We choose a trapping duration sufficiently short (Δ t =100 μs) to avoid shelving into the | D › manifolds currently limiting the lifetime at U max to milliseconds. To demonstrate optical trapping, we compensate the stray electric field to a level of ~80 mV m −1 only. The corresponding electric force results in a threshold for the critical optical potential U crit depicted as the vertical dashed line. Applying our novel compensation method to its current limitation of 8.7 mV m −1 (see text) will allow us to further reduce the laser power of the dipole beam and to increase the lifetime of the ion substantially. The vertical error bars denote the statistical error (1 σ ) of the respective measurement. Full size image For optimized conditions, for example, optimizing the initial laser cooling at U tot = k B × 55 mK, we currently reach optical trapping probabilities of up to (98±2)% (red diamond). The corresponding harmonically approximated oscillation frequency amounts to ω y ≈ ω z ≈2 π × 130 kHz. As a lower bound for the average time between two off-resonant events of photon absorption out of the dipole beam [42] , we estimate a coherence time of t coh =0.7 ms. We experimentally confirm the scattering rate 1/ t coh ≈1.4 × 10 3 s −1 by measuring the rate of electron shelving into the manifolds of the | D 5/2 › level. The branching ratio for the decay from the | P 3/2 › into the | S 1/2 › and the | D 5/2 › states amounts to 3:1. Two photon recoils of one absorption and emission event cause an energy transfer on the level of k B × 0.6 μK. In comparison with former results on optically trapping Mg + ions reported in ref. 34 , with a related scattering rate of 7.5 × 10 5 s −1 and a recoil energy of k B × 10 μK, we achieve a suppression of the recoil heating rate by four orders of magnitude. a.c. Stark shift-assisted stray electric field compensation To improve optical trapping of ions by further reducing the off-resonant scattering and improving coherence times seems straightforward. Following the established protocol for neutral atoms [42] , this involves increasing the detuning and the power of the dipole laser while reducing the initial temperature of the ion, in a first step down to the Doppler cooling limit at T D =300 μK. However, in contrast to optically trapped neutrals, ions feature the additional charge directly coupling to electric fields, making them prone to stray electric fields and forces [43] . We have to overcome these by optical means, that is, to counteract by the gradient of the optical potential ( ∝ ∇ I ). Thus, to improve the performance of optical ion traps, it remains a fundamental prerequisite to further enhance the capability to compensate stray electric fields. We present a novel method for stray electric field compensation, applicable for many ion species and any trapping potential, demonstrated for a Ba + ion confined by the electric fields of a linear Paul trap. For this purpose, we employ our tightly focused, attenuated dipole beam ( P ≈1 W) to probe the position of the ion. The intensity profile causes a spatial dependency of the a.c. Stark shift of the ion’s electronic levels, of the related detuning of our detection laser and therefore of the fluorescence rate. Ideally, even a significant change of the rf confinement should not affect the position of the minimum of the rf potential. However, because the ion is exposed to a stray electric field E S , it is displaced to the minimum of the total potential. Here it is given by the superposition of rf and d.c. fields. Consequently, switching between two extremal rf amplitudes—that is, between the maximal and minimal secular frequencies that are still providing stable confinement—leads to two distinct locations of the ion probing different a.c. Stark shifts. The related change of fluorescence then permits to derive E S . To apply our method, we detect the fluorescence of an ion in the rf trap by driving the cooling and repumping transitions while performing the following protocol (see Fig. 3 ): 1 We employ a procedure for pre-compensation consisting of a coarse version of the protocol for fine tuning described below. Here, we minimize the fluorescence rate directly on the CCD (charge-coupled device) camera. First, at maximal rf confinement (currently at ω y =2 π × (307±0.1) kHz), we coarsely centre the dipole beam on the ion using micrometre screws on the objective mount (see Fig. 3a ). Second, we switch to minimal rf confinement (currently ω y =2 π × (27.3±0.1) kHz). Now we minimize the related displacement of the ion by applying d.c. potentials to the compensation electrodes to shift the ion back to its original position again (for details see the Methods section). 2 We derive the profile at the centre of the dipole beam (again at maximal rf confinement) and overlap it with the ion. That is, we probe the fluorescence in dependence of 91 piezo-controlled positions of the attenuated dipole beam. We then reveal its profile via a quadratic fit (see Fig. 4 ) and centre it again on the ion now according to the fit with the accuracy of the piezo actuators (see Fig. 3a ). Figure 4: Measurement of the profile of the dipole beam. 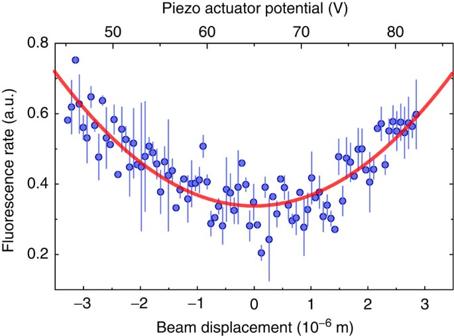Figure 4: Measurement of the profile of the dipole beam. Fluorescence rate of an ion trapped in an rf field providing maximal confinement (ωy=2π× (307±0.1) kHz) in dependence on the potential applied to the piezo actuators and the displacement of the centre of the dipole beam along they-direction, respectively. The dipole beam is inducing an a.c. Stark shift on the electronic energy levels of the ion, increasing the detuning of the cooling laser from the atomic transition and, thus, decreasing the fluorescence rate. The dependence of fluorescence in the vicinity of the centre of the (Gaussian shaped) dipole beam, is approximated quadratically and its centre determined by a least square fit (solid line) with an uncertainty of 26 nm. The vertical error bars denote the statistical error after an integration time of 1 s per data point (1σ). Fluorescence rate of an ion trapped in an rf field providing maximal confinement ( ω y =2 π × (307±0.1) kHz) in dependence on the potential applied to the piezo actuators and the displacement of the centre of the dipole beam along the y -direction, respectively. The dipole beam is inducing an a.c. Stark shift on the electronic energy levels of the ion, increasing the detuning of the cooling laser from the atomic transition and, thus, decreasing the fluorescence rate. The dependence of fluorescence in the vicinity of the centre of the (Gaussian shaped) dipole beam, is approximated quadratically and its centre determined by a least square fit (solid line) with an uncertainty of 26 nm. The vertical error bars denote the statistical error after an integration time of 1 s per data point (1 σ ). Full size image 3 We measure the displacement of the ion along the y axis due to switching of the rf confinement to its minimum amplitude (see Fig. 3b ). That is, we keep the dipole beam at the position set in step 2 and probe the fluorescence in dependency of the d.c. potentials applied to the (compensation) electrodes of the trap (see Fig. 5 ). Figure 5: Fluorescence rate of an ion in dependence on the electric field. 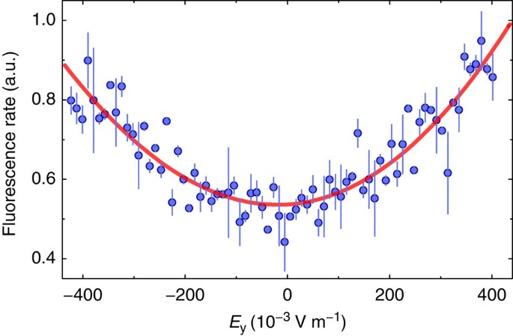Figure 5: Fluorescence rate of an ion in dependence on the electric field. Ey(along they-direction) is caused by the potential applied to the trap electrodes. The ion probes the intensity profile of the dipole beam in the vicinity of its centre. The centre of this beam profile can be approximated by a least square fit of a quadratic function with an uncertainty of 6.0 mV m−1(solid line). The potential at the electrodes can be calibrated to an electric field, as described in the Methods section, with a relative error of 11%. The vertical error bars denote the statistical error (1σ) of the fluorescence rate. E y (along the y -direction) is caused by the potential applied to the trap electrodes. The ion probes the intensity profile of the dipole beam in the vicinity of its centre. The centre of this beam profile can be approximated by a least square fit of a quadratic function with an uncertainty of 6.0 mV m −1 (solid line). The potential at the electrodes can be calibrated to an electric field, as described in the Methods section, with a relative error of 11%. The vertical error bars denote the statistical error (1 σ ) of the fluorescence rate. 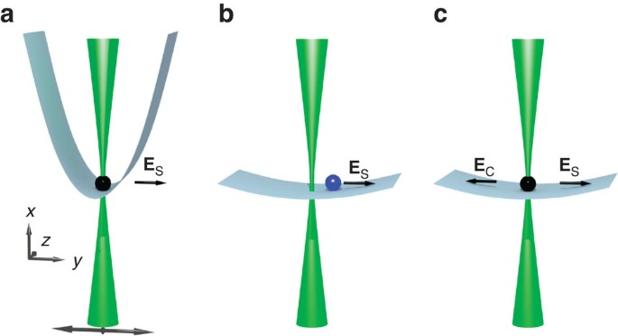Full size image 4 We derive the displacement of the ion from the centre of the beam profile via a quadratic fit and adjust the compensation field, E C , by the appropriate d.c. potential to recentre the ion (see Fig. 3c ). Figure 3: Schematic of the procedure to compensate a stray electric field ES. Our scheme is based on exploiting the a.c. Stark shift induced by a tightly focused dipole laser beam (green) as well as the related modulation of the fluorescence rate of the ion exposed to a detection beam (not shown). The latter is tuned close to the unshifted transition and of nearly constant intensity on the scale of relevant displacements. (a) The dipole beam is first characterized and centred on the ion (black sphere) at maximal confinement (ωy=2π× (307±0.1) kHz). This is done by displacing the beam along a chosen axis (hereyaxis) with micrometre screws (see step 1 in the main text) and piezo actuators (see step 2 in the main text andFig. 4) respectively, as indicated by the double-headed arrow at the bottom. (b) The confinement is switched to its minimal value (ωy=2π× (27.3±0.1) kHz) and the ion (blue sphere) shifts into the new equilibrium position at lower intensity of the dipole laser beam. Thus, with its transition closer to resonance with the detection beam, this leads to increased fluorescence. (c) The ion is moved to its original position inawith the compensation fieldECinduced by potentials applied to compensation electrodes along theyaxis (see steps 3 and 4 in the main text andFig. 5). Figure 3: Schematic of the procedure to compensate a stray electric field E S . Our scheme is based on exploiting the a.c. Stark shift induced by a tightly focused dipole laser beam (green) as well as the related modulation of the fluorescence rate of the ion exposed to a detection beam (not shown). The latter is tuned close to the unshifted transition and of nearly constant intensity on the scale of relevant displacements. ( a ) The dipole beam is first characterized and centred on the ion (black sphere) at maximal confinement ( ω y =2 π × (307±0.1) kHz). This is done by displacing the beam along a chosen axis (here y axis) with micrometre screws (see step 1 in the main text) and piezo actuators (see step 2 in the main text and Fig. 4 ) respectively, as indicated by the double-headed arrow at the bottom. ( b ) The confinement is switched to its minimal value ( ω y =2 π × (27.3±0.1) kHz) and the ion (blue sphere) shifts into the new equilibrium position at lower intensity of the dipole laser beam. Thus, with its transition closer to resonance with the detection beam, this leads to increased fluorescence. ( c ) The ion is moved to its original position in a with the compensation field E C induced by potentials applied to compensation electrodes along the y axis (see steps 3 and 4 in the main text and Fig. 5 ). Full size image Depending on the amplitude of the initial stray electric field E S , we have to consider its initial impact on the derivation of the centre of the rf trap in step 2. It leads to a systematic error, positioning the ion at the centre of the total potential. However, this error can be mitigated by iterating our protocol (steps 2–4). Currently, we estimate an upper bound for the uncertainty of the residual electric field of Δ E S ≈8.7 mV m −1 . A more detailed treatment of the remaining systematic errors and the limitations is given in the Discussion and Methods section. To benchmark our current results, we compare them with those achievable by state-of-the-art techniques in rf traps for different applications, featuring a minimal electric field uncertainty in the range of a few 100 mV m −1 (for example, see ref. 18 ), and with specific experimental arrangements 20 mV m −1 (ref. 44 ). Owing to our improvements, even in hybrid traps, the achievable compensation level is within the limits that are predicted to be sufficient to enter the s-wave regime—at least for the few selected ion–atom combinations not being practically excluded already. This applies for ensembles restricted to constituents with the largest ion–atom mass ratios, such as Li and Yb + (ref. 20 ). The method is additionally advantageous, especially for optical traps for ions, because it optimizes the spatial overlap between the optical and the initializing rf trap as well. It therefore mitigates the gain in the potential energy of the ion caused by the not fully adiabatic transfer between the traps. In summary, it allows further reduction of the required critical intensity of the optical trapping beam by more than a factor of 10 compared with the compensation level used for the optical trapping experiments described above (see Fig. 2 ), further prolonging the coherence time accordingly. To take full advantage of the decreased (critical) potential depth U crit , we will improve laser cooling to reach the standard Doppler limit at 300 μK and optionally increase the repumping efficiency [45] to keep the ion in the | S › manifold. To take our method to the limits set by state-of-the-art technology, we propose the following improvements. First, decreasing the position uncertainty by further reducing W of the diagnostics beam (dipole beam at low intensity) or by implementing a standing wave with a λ /2-periodic intensity pattern [46] decreasing the uncertainty of the electric field Δ E S by a factor of 2 W / λ ≈16. Second, increasing the reproducibility of the piezo-control of the beam position by a factor of 100 by state-of-the-art equipment, which should result in Δ E S <1 mV m −1 , otherwise, to the best of our knowledge, approached only by exploiting Rydberg atoms [47] , a method incompatible with rf fields. At this level and for a setup suited for trapping ions, we expect another class of systematic effects to affect the precision of our method, such as thermal expansion of and drifting potentials at the electrodes (see Methods). However, we emphasize that statistical fluctuations, such as beam pointing of the dipole laser or generic vibrations in the setup, lead to a symmetric broadening of the fluorescence signal and a reduced sensitivity, but do not result in systematic errors. To address all spatial degrees of freedom a second dipole laser beam is advantageous. For our current application of choice, this can be achieved, for example, by exploiting a crossed beam arrangement common in all-optical BEC experiments [48] . To put the current results of the suppressed photon scattering and stray field uncertainty in a relevant perspective, we consider the prospects for experiments of optically trapped ions immersed in a bath of ultracold atoms. To achieve efficient (sympathetic) cooling and to reach nanokelvin temperatures by elastic scattering of the ion with ultracold atoms [33] , we have to compare the residual recoil heating rate due to off-resonant photon scattering with the (in)elastic scattering rate between Ba + and Rb, responsible for the sympathetic cooling (chemical reaction). Already at our current level of stray field compensation and reduced power required in the dipole beam, on the order of 100 undisturbed elastic scattering events should take place [26] before the first occurrence of a photon recoil event. The latter is responsible for disrupting coherent processes and limiting sympathetic cooling. The rate for inelastic collisions is suppressed by another factor of ~10 4 (ref. 33 ). We estimate that we require a few (<10) collisions to allow for sympathetic cooling to the temperature of equilibrium with the atomic bath [49] , thus recoil heating remains negligible. Consequently, the current realization is already sufficient for exemplary applications: first, to study ultracold interactions, for example, the potential formation of mesoscopic clusters [32] , and second, to extend and alter the recently achieved breakthrough in studying long-range interaction in homonuclear systems of Rydberg atoms within BECs [50] . On the other hand, the inelastic (incoherent) processes, such as molecule formation in the quantum regime of s-wave scattering are of interest in their own right [22] , [23] , [24] , [25] , [26] , [33] . In our current implementation, the trapping laser at 532 nm remains blue detuned with respect to the transitions between the electronic | P › and the metastable | D › states of Ba + . For our envisioned application, shelving into the sublevel manifolds of the | D › states is not desirable, since the related deconfinement leads to shorter lifetimes of the ion and thus derogates statistics. There are several options to minimize or mitigate this effect. First, an additional, farther detuned, laser (of a bichromatic trap) at 1,064 nm—initially mainly responsible for the optical trapping of Rb—can also be used to simultaneously trap Ba + (switching off the 532 nm beam after sympathetic and evaporative cooling). At sufficiently low temperatures, such substantially increased detuning should make it possible to confine the ion in the | S › and | D › states simultaneously (red detuned with respect to both transitions). Second, already implemented laser beams at 615 and 650 nm can be used to resonantly repump the population into the electronic ground state. Optionally, the dependence of the detuning on the spatially modulated a.c. Stark shift can be mitigated by interchangeably exposing the ion to the dipole and the repumping beams at a rate high compared with the secular frequency within the optical potential. Third, as an alternative approach, tuning the frequency of the dipole laser blue of resonance, in combination with confining d.c. fields, might allow us to further reduce off-resonant excitation while providing trapping in | S › and | D › manifolds simultaneously. Initial coarse compensation of stray electric fields To mitigate the systematic error related to the initial displacement of the ion from the node of the rf potential in presence of the finite stray electric field, we employ step 1 of the compensation protocol described in the main text before performing protocol steps 2–4. This preparatory procedure with a total duration of ~60 s has to be carried out approximately once a day. We note that iterating steps 2–4 of the described scheme without the preparatory step 1 allows us to compensate within a measurement duration of n times 167 s, to a level of |Δ E S |=8.7 mV m −1 or lower. This precision can also be reached after a single cycle if we compensate the initial stray electric field to or below. To this end, it is sufficient to locate the rf node with an uncertainty of approximately W y /2 at maximum rf confinement and subsequently position the ion within this distance at the dipole beam centre at minimal rf confinement. Both procedures are confirmed by a readily detectable drop of the fluorescence rate to ~50%, respectively. The corresponding positioning errors with the chosen secular frequencies of ω y =2 π × (307±0.1) kHz and ω y =2 π × (27.3±0.1) kHz and a waist of W y =4 μm amount to . Uncertainty in the compensation of stray electric fields We assume that the electric field has already been compensated to the level of as described above (see Fig. 3 ). At maximal confinement ( ω y =2 π × (307±0.1) kHz), results in an initial displacement of d res ≈26 nm. In addition, the position of the centre of the dipole beam is estimated as the s.e. (1 σ ) of the least square fit (see Fig. 4 ) to d fit =56 nm. The dipole laser beam is shifted to discrete locations with a piezo-actuated mirror that can be reproducibly positioned with an uncertainty of d rep =94 nm with a minimal incremental step size of 2 nm. These uncertainties are added quadratically: . At the minimal confinement of ω y =2 π × (27.3±0.1) kHz, this yields an uncertainty of the residual electric field of Δ E align ≈4.6 mV m −1 . The uncertainty of centring the ion in the dipole trapping beam via potentials on compensation electrodes is obtained from the s.e. of the least square fit amounting to Δ E pos ≈6.0 mV m −1 (1 σ , see Fig. 5 ). The pointing of the beam, controlled by the piezo-mounted mirror, is drifting systematically during the measurements, which take ≈91 s for the laser alignment in step 2 and ≈76 s for the field compensation in step 4. We measure a corresponding drift rate of 0.5 nm s −1 and, without correcting for such systematic drifts after performing steps 2 and 4, assume that they simply accumulate. These drifts then lead to Δ E sys1 ≈0.9 mV m −1 and Δ E sys2 ≈0.7 mV m −1 , respectively. Thus, as a worst-case scenario, we estimate the total electric field uncertainty Δ E S by linearly adding statistic and systematic errors to . The impact of other systematic effects has been mitigated considering the argument presented in the following. First, the effect of light pressure of the cooling light on the ion can lead to significant displacement, and consequently to misalignment of the dipole beam. To minimize light forces along the y axis, we currently provide efficient cooling along the z - and x -direction only. In the future we will implement pairs of counter-propagating beams to provide optimal cooling towards the Doppler limit while additionally eliminating the net light pressure in all degrees of freedom. Second, effects of dipole forces induced by the dipole beam are minimized by substantially attenuating the dipole trapping beam. Third, the effects of thermal drifts of the trap geometry due to changes in rf amplitude are still negligible. On the basis of conservative estimates and measurements of the temperature, we conclude that the rf electrodes do not warm up by >0.3 K, corresponding to an upper bound for a spatial drift of the electrodes of 10 nm. Calibration of the electric field We derive the amplitude of the electric field provided at the position of the ion by calibrating the potential applied to the appropriate pair of rf electrodes to the ion displacement at a confinement of ω y =2 π × (307±0.1) kHz. We start by moving the dipole beam across the position of an ion in the rf trap. We verify that the induced a.c. Stark shift Δ S is smaller than the natural linewidths of the | S 1/2 ›←| P 1/2 ›, | P 3/2 › transitions of the ion and derive the beam waist W y along the y axis. A displacement of the beam by W y in a harmonic potential with a secular frequency of ω y requires a force , m being the mass of the ion. It can be related to an electric field E C along y with F y = eE C , where e is the elementary charge. Subsequently, we keep the laser beam fixed and move the ion along the y -direction by applying a potential V y to the corresponding electrodes. The recorded fluorescence pattern can be fitted by a Gaussian beam intensity profile yielding its width in units of the applied potential and, thus, the electric field E C . The calibration of the electric field to an applied potential is in agreement with numerical simulations using a finite difference method. The uncertainty of the residual stray field of Δ E S =8.7 mV m −1 is equivalent to an electric potential uncertainty of 19 μV on two adjacent electrodes. Optical trapping of Ba + in a far-off-resonance trap To derive the total trap depth U tot depicted in Fig. 2 , we perform a Monte Carlo simulation where we consider the centre of the dipole trap beam ( y 0 ), its waist ( W y ), the d.c. harmonic frequency ω y and the residual stray electric field Δ E S to be normally distributed. From 5 × 10 4 randomly generated values for the relevant variables, we numerically calculate the total trap depth along the y -direction (the direction with a repulsive d.c. potential, see Fig. 1 ) by determining the difference between the minimum and the smallest local maximum of the trapping potential where U 0 is the depth of the optical trapping potential [42] . By binning the values of U tot we obtain the probability distribution for the total trap depth and thus the mean value as depicted in Fig. 2 , as well as the corresponding s.d. To obtain the temperature from the optical trapping probability (see Fig. 2 ) for a given U tot , we consider the radial cutoff model introduced in ref. 35 with ξ = U tot /( k B T ), where we assume all heating rates such as recoil and anomalous heating (see below) to be negligible for the duration of the optical trapping. The optical confinement along the focal direction ( x axis) of the dipole trap is weak compared with the confinement along the y - and z -axes. We provide additional d.c. confinement along the x axis, which we achieve by tilting the principle axis with an accuracy of ±25° with respect to the laboratory frame resulting in a bare d.c. confinement with , and . Potential influence of anomalous motional heating Anomalous heating is a major concern for the field of trapped ions that attracted and still attracts a substantial amount of attention in the community [51] , [52] . However, anomalous heating mainly affects the perspective for the miniaturization of rf traps, since this heating rate scales with R −4 , R standing for the distance between the ion and the electrodes. Fortunately, we have to scale the size of our apparatus in the opposite direction, since we are even dependent on large R for our approach to optical trapping of ions and large ensembles of atoms. Thus, the contribution from anomalous heating is expected to be small compared with other sources of decoherence, such as recoil heating. To obtain a quantitative estimate of this contribution, we perform a measurement of the heating rate based on resolved sideband spectroscopy via two-photon-stimulated Raman transitions. Owing to limitations of the optical access in the apparatus described here, these measurements have been carried out in a similar setup particularly equipped for this purpose, which was recently used to demonstrate optical trapping of Mg + ions, with R 1 =0.4 mm. We start by cooling a Mg + ion close to the motional ground state and evaluate the ratio of the transition amplitudes of the first red and blue sidebands, yielding a mean vibrational quantum number of . To obtain a heating rate, we perform this procedure for different delay periods between preparation and detection. We find a motional heating rate of quanta per second at a secular frequency of ω sec =2 π × 2 MHz and quanta per second at a secular frequency of ω sec =2 π × 1 MHz corresponding to a heating rate of ~1.5 × 10 −3 K s −1 . With an ion–electrode spacing of R 2 =1.12 mm in the current setup and already considering the decreased secular frequencies, we estimate a heating rate of 2.4 × 10 −5 K s −1 . We find that the expected heating rate is negligible, even assuming such a conservative scenario and in absence of any cooling mechanisms. We note that in ultracold ion–atom (for example, Ba + and Rb) collision experiments in absence of micromotion, sympathetic cooling of the ions is expected to dominate with an estimated rate on the order of 10 −2 K s −1 . Furthermore, the apparatus designed for the proposed experiment features R 3 =8 mm. Thus, it remains highly unlikely that anomalous motional heating can affect our envisioned results, even assuming an unfavourable scaling of the noise spectrum. However, if optical ion trapping is considered in combination with miniaturized or even surface electrode traps in the future, aiming, for example, to implement more complex (and shallower) optical lattice potentials and ion arrays or ions and atoms stored in neighbouring lattice sites, the contributions from anomalous heating might have to be actively addressed. To this end, several approaches have been established for further suppressing heating rates, such as electrode surface cleaning [52] or cryogenic environments [51] . How to cite this article : Huber, T. et al. A far-off-resonance optical trap for a Ba + ion. Nat. Commun. 5:5587 doi: 10.1038/ncomms6587 (2014).